Resonance shifts and spill-out effects in self-consistent hydrodynamic nanoplasmonics The standard hydrodynamic Drude model with hard-wall boundary conditions can give accurate quantitative predictions for the optical response of noble-metal nanoparticles. However, it is less accurate for other metallic nanosystems, where surface effects due to electron density spill-out in free space cannot be neglected. Here we address the fundamental question whether the description of surface effects in plasmonics necessarily requires a fully quantum-mechanical ab initio approach. We present a self-consistent hydrodynamic model (SC-HDM), where both the ground state and the excited state properties of an inhomogeneous electron gas can be determined. With this method we are able to explain the size-dependent surface resonance shifts of Na and Ag nanowires and nanospheres. The results we obtain are in good agreement with experiments and more advanced quantum methods. The SC-HDM gives accurate results with modest computational effort, and can be applied to arbitrary nanoplasmonic systems of much larger sizes than accessible with ab initio methods. Many recent experiments on dimers made from closely coupled metallic nanoparticles and other nanoplasmonic structures have revealed phenomena that require to go beyond classical electrodynamics for their description. To explain these new phenomena, a unified theory would be highly desirable that includes nonlocal response, electronic spill-out as well as retardation. And ideally such a theory would lead to an efficient concomitant computational method. To his end, one could try to generalize standard density-functional (DFT) theory to include retardation or to generalize standard hydrodynamic theory so as to include free-electron spill-out at metal–dielectric interfaces. In this work we present the latter, both the generalized hydrodynamic theory and its efficient numerical implementation. The hydrodynamic Drude model (HDM) of the electron gas is one of the most commonly used methods for the computational study of plasmonic nanostructures beyond classical electrodynamics [1] . This model has been used in recent years to determine the optical response of coupled nanoparticles [2] , [3] , [4] , [5] , [6] , [7] , [8] , [9] , [10] , [11] , [12] , the limitations on field enhancement in subwavelength regions [13] , [14] , the nanofocusing performances of plasmon tips [15] and the fundamental limitations of Purcell factors in plasmonic waveguides [16] . The most important feature of this model is its ability to describe the plasmonic response of noble-metal nanoparticles at size regimes at which the classical Drude metal is no longer valid, with a high accuracy and a low computational effort. This is obtained by including the Thomas–Fermi pressure in the equation of motion of the electron gas [1] that takes into account the fermion statistics of the electrons. The HDM provides accurate predictions of the spectral positions of the surface-plasmon resonances (SPRs) for noble-metal dimers and for single particles it mimics the SPR blueshift that grows as the particle size decreases. In line with the local-response Drude model, the standard implementation of the HDM usually considers the so-called hard-wall boundary condition, that implies that the electrons are strictly confined in the metallic structure, with a uniform equilibrium density and without spill-out in free space [1] . This approximation is more accurate for noble metals, that show a high work function [17] , than for alkali metals [18] , [19] , [20] , [21] , where the electron density spill-out in free-space characterizes the plasmonic response. This is a well-known limitation of the HDM [22] and many attempts have been made to overcome it, thus far with limited success. In a pioneering attempt, Schwartz and Schaich [23] proposed to relax the hard-wall constraint by introducing equilibrium electron density distributions obtained with different methods in the hydrodynamic equations. They found that continuous surface densities lead to the proliferation of spurious surface multipole modes, qualitatively disagreeing with experimental results, which lead them to conclude that the HDM approach to surface effects is subject to a considerable uncertainty. In a recent work, David and García de Abajo [12] showed that a better agreement between the HDM results and experimental data can be obtained if an equilibrium electron density from DFT calculations is employed. However, the issue of whether the hydrodynamic model per se is a valid theory to describe surface effects in plasmonic nanostructures is still open. At present, one is lead to believe that the ground state properties of an electron system must be always calculated by means of refined ab initio methods. A hint towards the solution of this problem can be found in a seminal paper by Zaremba and Tzo [24] on the hydrodynamic theory of inhomogeneous systems. In this work, the authors point out that the equilibrium density of the electrons in a metal cannot be chosen arbitrarily, but it must be calculated self-consistently within the hydrodynamic theory itself. Any failure to do so would lead to spurious solutions, as in the case of Schwartz and Schaich’s work [23] . Inspired by this observation, we introduce a self-consistent hydrodynamic model (SC-HDM) for the inhomogeneous electron gas. In this context, both the ground state and excited state properties of a generic electronic system can be determined and hard-wall or other additional boundary conditions at the metal–dielectric interface are no longer needed. We apply this method to the study of the optical response of alkali (Na) and noble-metal (Ag) nanowires, because sodium nanowires were recently used as an example to illustrate the lack of accuracy of standard hydrodynamic theory [20] , [21] . By contrast, without any fitting and without heavy computations we obtain with our self-consistent hydrodynamic method accurate agreement both with experiments and with more advanced theories. This illustrates the promising use of our self-consistent hydrodynamic method in nanoplasmonics, where efficient methods that take into account retardation, nonlocal response as well as spill-out are highly demanded but scarce. We also show that similar results can be obtained for three-dimensional (3D) particles while discussing the spectral response from Na and Ag nanospheres. Hydrodynamic equations We first briefly recall how in general hydrodynamic equations are derived in terms of functional derivatives of the internal energy of an electron plasma, before specifying our choice for the internal energy. The Bloch hydrodynamic Hamiltonian for the inhomogeneous electron gas [25] reads: where n ( r , t ) is the electron density and p ( r , t )= m v ( r , t )+ e A ( r , t ) its conjugate momentum, with e being the electron charge and m the electron mass. The electrons are coupled to the electromagnetic field associated with the retarded potentials φ ( r , t ) and A ( r , t ), that is, and B ( r , t )= ∇ × A ( r , t ). The electrostatic potential V back ( r ) is a confining background potential, that is associated with the electrostatic field generated by the positive ions in a metal, that is, ∇ 2 V back ( r )=− ρ + ( r )/ ɛ 0 , where ρ + ( r ) is the positive-charge density of the metal ions. The term G [ n ( r , t )] is the internal energy of the electron gas, which is assumed to be a functional of the electron density. Its functional form is not known a priori and we will specify and motivate our particular choice later. The equations of motion can be obtained from equation (1) by means of the methods of the Hamiltonian formulation of fluid dynamics [26] , [27] , [28] (see Supplementary Note 1, 2 and 8 ). The force balance on a fluid element is stated by the Euler equation (and in the following we will for simplicity suppress the ( r , t ) dependence) where the density n satisfies the charge continuity equation We focus on the linear response of the electron gas described by equation (1), so we solve equations (2) and (3) for small perturbations of the electron density n 1 ( r , t ) around the equilibrium density n 0 ( r ), that is, n ( r , t )= n 0 ( r )+ n 1 ( r , t ) [29] . It can be shown (see Supplementary Note 3 ) that n 0 ( r ) satisfies where φ 0 is the potential associated with the electrostatic field E 0 generated by the equilibrium charge density ρ 0 = en 0 . Thus φ 0 and ρ 0 are related by Poisson’s equation ∇ 2 φ 0 ( r )=− ρ 0 ( r )/ ɛ 0 . The quantity is the functional derivative evaluated at the equilibrium density n 0 , and μ represents the (constant) chemical potential of the electron gas. Equation (4) is quite general and also appears in standard DFT [30] , [31] . It is useful to write the linearized versions of both the force-balance equation (2) and the charge continuity equation (3) in terms of the electric-charge density perturbation ρ 1 = en 1 and the first-order electric current-density vector J 1 = en 0 v 1 ≡ ρ 0 v 1 . The linearized Euler equation for the current-density vector J 1 reads while the linearized continuity equation becomes The quantity in equation (5) is given by , and ω p =[ e 2 n 0 /( mɛ 0 )] 1/2 is the spatially dependent plasma frequency of the electron gas. The vector fields E 1 and J 1 satisfy Maxwell’s wave equation The linear system given by equations (5), (6) and (7) is closed, and can be solved once the equilibrium density ρ 0 ( r ) has been calculated by means of equation (4) (see Supplementary Note 3 and 4 ). It is important to notice that retardation effects due to time-varying magnetic fields are included in the system above, so that both longitudinal and transverse solutions are possible. This is an important difference with state-of-the-art time-dependent DFT (TD-DFT) methods, that only solve for longitudinal currents and electric fields [32] . The linearization procedure of the hydrodynamic equations that we have outlined so far is logically consistent, since no external assumptions on the quantities involved are required. In particular, rather than a postulated function, the static electron density n 0 ( r ) is a solution of equation (4). We call this method ‘SC-HDM’, to distinguish it from other implementations of the hydrodynamic model that import an equilibrium charge density that is not based on the same Hamiltonian for the system as the one used to calculate its linear response. And for our choice of the energy functionals as detailed below, we will be able to describe electronic spill-out, that is, a non-vanishing n ( r ) also outside the metal. Hydrodynamic Drude model With the purpose to clearly link the progress presented in this contribution to the state-of-the-art in nanoplasmonic simulations, we will shortly outline in the following how the ordinary HDM can be derived from the general hydrodynamic theory developed above. This is particularly useful to identify the approximations intrinsic in the ordinary HDM. We recall here the equation of motion for this model, that in the time domain reads [1] where β is called the hydrodynamic parameter, defined as and v F is the Fermi velocity, . In the usual implementations of the HDM, a uniform equilibrium electron density n 0 ( r )= n 0 is assumed and the electron density spill-out in free space is neglected. This leads to the hard-wall boundary condition, stating that the current-density vector J 1 has a vanishing normal component at the surface of the metallic nanostructures. For this reason, in the next sections we will refer to this model as ‘hard-wall hydrodynamic model’ (HW-HDM). It can be readily shown that equation (8) can be derived from equation (5), if we consider n 0 ( r )= n 0 inside the metal and approximate the internal energy G [ n ] by means of the Thomas–Fermi kinetic energy functional multiplied by a constant parameter α =9/5 that accounts for the high-frequency corrections [33] (see below the discussion about the choice of the energy functionals). Moreover, it is possible to prove that a uniform equilibrium electron density is a solution of equation (4), thus the HDM is a special case of the SC-HDM (see Supplementary Note 9 ). Finally, we would like to mention that if the hydrodynamic parameter β vanishes, equation (8) reduces to the Drude equation of motion for the free-electron gas. We call this well-known model ‘local-response approximation’ (LRA), since it neglects the nonlocal electromagnetic effects associated with the spatial derivative of the charge density ρ 1 in the equation of motion. Including density gradients in the energy functional After obtaining the closed system of linearized hydrodynamic equations, we now specify and motivate the form of the energy functional that features in them. The internal energy functional G [ n ( r , t )] in equation (1) is given, in general, by the sum of a kinetic energy functional T [ n ( r , t )] and an exchange-correlation (XC) energy functional F xc [ n ( r , t )] (ref. 31 ): In TD-DFT, the kinetic energy term T [ n ( r , t )] is calculated by means of the Kohn–Sham equations, a task that is computationally demanding for particles consisting of much more than 10 3 electrons, in other words for most experiments in nanoplasmonics. The main goal of our SC-HDM is therefore to provide an alternative computational tool for particles and structures of larger sizes and lower symmetry than TD-DFT currently can handle. We do this by means of an orbital-free (OF) approach [34] , [35] , [36] , [37] . Below we discuss the kinetic- and XC-energy functionals separately. We approximate the kinetic energy functional by the sum of the Thomas–Fermi functional and the von Weizsäcker functional [38] , Here the last term is the von Weizsäcker functional, which is also called the ‘second-order gradient correction’ to the Thomas–Fermi kinetic functional [30] . Such a gradient correction can become important in space regions where n 0 ( r ) shows strong variations, for example in the vicinity of metal surfaces as we shall see below, and especially when describing molecules [30] . Our choice is motivated by the fact that the T TFW functional is known to provide reliable descriptions of surface effects in metals, and it has been extensively employed in solid-state physics to calculate the work functions and surface potentials of various metals [39] , [40] , [41] , [42] , [43] . Although adding the functional T TFW will significantly improve the accuracy of hydrodynamic calculations, it will not reconstruct the wave nature of the electrons, inherent, for example, in the Friedel oscillations into the metal bulk, which require the full Kohn–Sham calculations with XC functionals [44] . In nanoplasmonics only the Thomas–Fermi functional was used until now [2] , [3] , [4] , [5] , [6] , [7] , [8] , [9] , [10] , [11] , [12] , [13] , [14] , [15] , [16] , while to our knowledge the second-order gradient correction has thus far been neglected. Below we will give an example where the calculations of optical properties based on only the Thomas–Fermi functional disagree with experiment, while agreement is found when including the von Weizsäcker functional, in combination with the XC functionals as discussed below. An exact expression for the XC functional is not known in general [30] , and it is not easy to calculate it numerically either, so an approximation of the F xc [ n ( r , t )] is commonly employed, for example for performing the TD-DFT calculations. The most familiar one is the local-density approximation (LDA), where the name implies that no density gradients are considered in the construction of the functional. Just like for the kinetic functional, gradient corrections to the XC functional may nonetheless become significant for inhomogeneous systems. This calls for non-local density approximations (NLDAs) beyond LDA, to correct for the long-range effects arising for strong density variations. On a par with our treatment of the kinetic functional, we will also include density gradients in the XC functional that enters our hydrodynamic equations. In particular, we include the Gunnarson and Lundqvist LDA XC functional [45] , that has been used both for Na refs 21 , 46 and Ag (ref. 47 ). In addition, we include a nonlocal correction (NLDA) for long-range effects, namely the van Leeuwen and Baerends potential (LB94; ref. 48 ), which has already been used for Ag and Au plasmonic nanostructures [49] , [50] . Incidentally, when leaving out the NLDA exchange term to the functional, we found non-physical solutions with density tails propagating in the free-space region. This is another argument, besides transparency, for requiring self-consistency: a physical solution of n 0 is a test whether the energy functional captures the essential physics. We only study linear response ( n 1 and so on) in a model that passes the test for n 0 . This anomalous behaviour of the solutions has also been reported by Yan in a very recent paper [51] , for a hydrodynamic model without NLDA corrections for long-range effects. More well-behaved solutions were obtained by parameter fitting of the von Weizsäcker term. This procedure is certainly valuable, but does not address the underlying reason of the problem of the unphysical solutions, that we think lies in neglecting the long-range XC effects [34] . With the above choice of the XC functionals, we for simplicity deliberately neglect Landau damping of the collective modes caused by electron–hole transitions. This sharpens the spectral linewidths of the plasmonic resonances but has only weak influence on resonance peak positions that we focus on here. Future studies to include Landau damping into the SC-HDM could use ref. 34 as a starting point. Hereby we have specified and motivated the total energy functional that we will employ in our hydrodynamic theory. The inclusion of the density-gradient terms will make the crucial difference with state-of-the-art hydrodynamic theory used in plasmonics. We will soon show predictions that agree well both with experiments and with more advanced theory. Finally, we want to emphasize that the choice of the functionals is not universal, and that the ones we used here are standard functionals employed in the literature for isolated metallic nanoparticles. For different systems, such as bimetallic nanoparticles or functionalized metallic surfaces, further refinements might be needed. These refinements can affect, for example, the XC functional, since the substantial freedom in the choice of this functional is a known issue for all DFT-based ab initio methods, including Kohn–Sham-based DFT. Nevertheless, the OF-DFT-based methods such as the SC-HDM, need further consideration, since they are based on a truncated expansion of the kinetic energy functional. In fact, this constitutes the only essential difference with TD-DFT. The study of more refined OF kinetic energy functionals adapted to specific systems is the focus of ongoing research [37] , [52] , [53] , [54] and the interest of the DFT community in this topic has been growing in the recent years. Implementation of the SC-HDM We implemented the SC-HDM with the finite-element method in the commercially available software COMSOL Multiphysics 4.2a. This is a pragmatic choice, motivated by the fact that COMSOL offers a quite flexible implementation of the finite-element method, which can also be easily adapted to solve the SC-HDM equations. However, other computational schemes could be adopted, and ad hoc solvers could in principle be developed (see Supplementary Note 6 ). Equation (4) is nonlinear in the electron density, and it can be easily implemented when the ionic background of the metallic system is specified. We employ the jellium model for the ions, a standard approximation that is also successfully adopted in state-of-the-art TD-DFT calculations [20] , [21] , [55] . The linear differential system given by equations (5) and (7) was transformed to the frequency domain. We then solved for the induced charge density ρ 1 instead of the induced current-density vector J 1 . This is numerically advantageous, since it allows to solve for only one hydrodynamic variable ( ρ 1 ) instead of the three components of J 1 . The full implementation procedure and the computational efficiency of the numerical code are discussed in detail in the Supplementary Note 4 and 5 . In the following we describe at first results of 2D nanowires and later present results for 3D structures. Optical response of sodium nanowires We apply our formalism at first to derive the optical response of a Na cylindrical nanowire of radius R =2 nm. In the first step of our analysis, we calculate the equilibrium electron density n 0 of the Na nanowire by means of equation (4). The positive background density of the jellium is given by the ion density of Na, that is, n + =2.5173 × 10 28 m −3 . The result is shown in Fig. 1b (dashed line). Besides the charge spill-out into free space, n 0 also exhibits an oscillation within the metal. This is somewhat reminiscent of Friedel oscillations, whereas true Friedel oscillations at wavelength λ F /2 with the correct envelope require solving the full Kohn–Sham equation with suitable XC functionals. 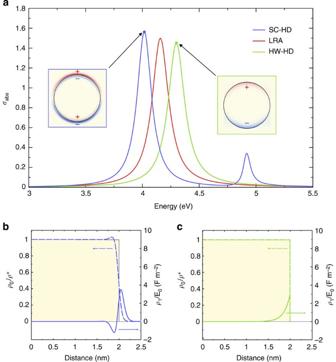Figure 1: Optical Response of a Na cylindrical nanowire of radiusR=2 nm. (a) Absorption cross-sectionσabsversus photon energy in the LRA (red line), the HW-HDM (green line) and the SC-HDM (blue line). The insets show the charge density distributionsρ1(r) at their respective dipolar SPR frequencies for the SC-HDM (blue box) and the HW-HDM (green box). (b) SC-HDM: equilibrium electron charge densityρ0normalized to the ion charge densityρ+(dashed line) and induced charge densityρ1normalized to the perturbing field amplitudeE0for the dipolar SPR, as a function of the distance from the axis of the nanowire. The light yellow shaded area indicates the jellium background profile. (c) As panel (b), now for the HW-HDM. Figure 1: Optical Response of a Na cylindrical nanowire of radius R =2 nm. ( a ) Absorption cross-section σ abs versus photon energy in the LRA (red line), the HW-HDM (green line) and the SC-HDM (blue line). The insets show the charge density distributions ρ 1 ( r ) at their respective dipolar SPR frequencies for the SC-HDM (blue box) and the HW-HDM (green box). ( b ) SC-HDM: equilibrium electron charge density ρ 0 normalized to the ion charge density ρ + (dashed line) and induced charge density ρ 1 normalized to the perturbing field amplitude E 0 for the dipolar SPR, as a function of the distance from the axis of the nanowire. The light yellow shaded area indicates the jellium background profile. ( c ) As panel ( b ), now for the HW-HDM. Full size image To determine the optical response of the system, we irradiate the nanowire with an in-plane polarized plane wave of amplitude E 0 =1 V m −1 , as in ref. 4 . All the perturbed quantities are calculated by means of the equation of motion (5), where a damping factor γ is introduced to take into account the electron–phonon interaction, dissipation due to the electron–hole continuum, impurity scattering and so on. We choose the value ℏ γ =0.17 eV from ref. 56 . Interband effects are not included, since for Na their effects in the visible range are negligible [57] . The optical quantity that we consider is the absorption cross-section per unit length σ abs , defined as , where is the power density of the perturbing field. We compare the prediction by the SC-HDM with both the HW-HDM and with the usual LRA. The hydrodynamic parameter β for the HW-HDM is , where the Fermi velocity for Na is v F =0.82 × 10 6 ms −1 . The results are shown in Fig. 1a . The main SPR within the LRA occurs at ℏ ω res =4.158 eV. This resonance is blueshifted by 0.139 eV to become ℏ ω res =4.297 eV in the HW-HDM. In stark contrast, for the SC-HDM the resonance appears at ℏ ω res =4.017 eV, in other words redshifted by 0.141 eV with respect to the LRA. Apart from their different peak positions, the three SPRs in the absorption cross-section in Fig. 1a also exhibit different peak heights in the three models. An intuitive explanation for this behaviour can be provided on the basis of the different geometrical cross-sections in the three models: in the SC-HDM the electrons spill out from the surface of the nanowire, so the structure appears bigger than in the LRA. In contrast, the free electrons are pushed inwards into the metal in the HW-HDM, so this structure looks smaller than in the LRA. The redshift of the surface-plasmon resonance in Na is linked to the electron spill-out in free space, or more precisely, to the fact that the centroid of the induced charge density ρ 1 associated with the SPR is placed outside the jellium edge [19] , [21] , [58] . Our self-consistent calculations correctly reproduce this feature of ρ 1 at the SPR peak, as it is shown in Fig. 1b (solid line). This plot highlights a peak of ρ 1 in the free-space region and a dip in the internal region where the equilibrium density takes its maximal value. We normalized the induced charge density ρ 1 with respect to E 0 , since in the considered linear-response regime the induced charge density is linearly proportional to the amplitude of the applied field. To further confirm the validity of our method, we would like to stress that the spectral position ℏ ω res =4.017 eV of the SPR that we obtained within our semi-classical hydrodynamic theory, is in good agreement with the values obtained with TD-DFT methodologies for similar systems [20] , [21] . A perfect agreement is not achievable because of the different approximations that are intrinsic to each specific method (see Supplementary Note 7 and Supplementary Fig. 2 ). The absorption cross-section spectrum in Fig. 1a shows another resonance peak at ℏ ω res =4.918 eV. This resonance is known in the literature as ‘multipole surface plasmon’ or ‘Bennett resonance’, first predicted by Bennett in 1970 (ref. 59 ). The charge distribution ρ 1 associated with this resonance is characterized by the fact that its integral along a direction orthogonal to the surface vanishes identically [60] (see Fig. 2 ). The Bennett resonance is not observable in the LRA and HW-HD models in Fig. 1 , since it is an effect of the non-uniform charge density in the metal and the electron spill-out in vacuum [59] . We would like to point out that also in this case the spectral position of the Bennett resonance that we find is in the same range of the results obtained with other methods [20] , [21] , [58] , [59] , [61] . 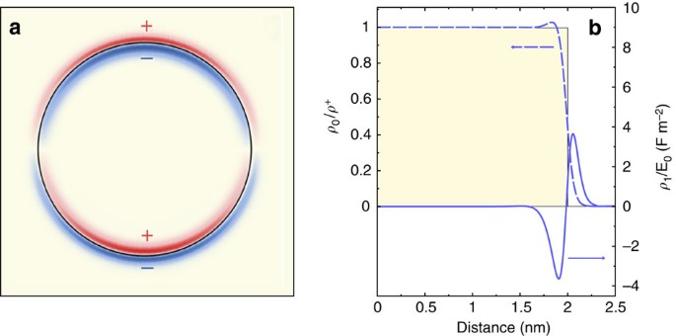Figure 2: Bennett resonance of a Na cylindrical nanowire of radiusR=2 nm. (a) Charge density distributionρ1(r). (b) Equilibrium electron charge densityρ0normalized to the ion charge densityρ+(dashed line) and induced charge densityρ1normalized to the perturbing field amplitudeE0for the Bennett SPR, as a function of the distance from the axis of the nanowire. The light yellow shaded area indicates the jellium background profile. Figure 2: Bennett resonance of a Na cylindrical nanowire of radius R =2 nm. ( a ) Charge density distribution ρ 1 ( r ). ( b ) Equilibrium electron charge density ρ 0 normalized to the ion charge density ρ + (dashed line) and induced charge density ρ 1 normalized to the perturbing field amplitude E 0 for the Bennett SPR, as a function of the distance from the axis of the nanowire. The light yellow shaded area indicates the jellium background profile. Full size image Figure 1c shows again an equilibrium electron density n 0 and an induced charge density ρ 1 , but now for the HW-HDM. Consistent with the hard-wall assumption, all charges in Fig. 1c are indeed localized inside the metal. The equilibrium density n 0 is constant and equal to the local-response value for bulk Na, whereas the induced density ρ 1 can be seen to decrease monotonically away from the surface, where in local response (not shown) all induced charge would reside in a delta-function distribution on the interface. Finally, a comparison of Fig. 1b,c nicely illustrates that the non-monotonous equilibrium and induced charge densities in the metal region and the spill-out in the air region are a consequence of taking density gradients into account in the energy functional of our self-consistent hydrodynamic theory. Optical response of silver nanowires We will now compare the optical response of Ag nanowires with that of Na nanowires as discussed above. The aim is to show that our self-consistent HD theory for both the types of metals agrees with experiment and with TD-DFT calculations. The free-electron gas in Ag consists of electrons in the 5s-band. Analogous to the case of Na that we discussed above, their spatial equilibrium distribution n 0 can be calculated within the jellium approximation for the positive-charge background. Such calculations of n 0 have already been done for noble metals, in DFT calculations for example [47] , [55] , [58] . However, unlike for Na, for Ag the interband transitions from the filled 4d-band to the 5s-band near the Fermi level often cannot be neglected in the optical response, so that Ag cannot be described as a pure Drude metal at optical frequencies. Because of this well-known fact, we will take interband transitions into account in our SC-HDM for Ag. In principle, a full-electron calculation could be used to account for interband transitions. However, this is computationally very demanding and beyond the aims and scope of our hydrodynamic approach. For this reason, we follow the prescription proposed by Liebsch [58] , treating the 4d-core electrons as an effective polarizable medium that contributes to the optical response by means of an interband permittivity ɛ inter . This medium is assumed to extend up to the first plane of the nuclei. In the jellium model, the distance d between the edge of the positive background and the first plane of nuclei amounts to half a lattice spacing, and this parameter can be obtained from experimental data on the specific metallic system. For example, in the case of the Ag (111), (001) and (110) faces, d is equal to 1.18, 1.02 and 0.72 Å, respectively [58] . For a good comparison, we again study nanowires of radius R =2 nm that are irradiated by a plane wave with in-plane polarization and amplitude E 0 =1 V m −1 . For Ag the ion density is n + =5.8564 × 10 28 m −3 , corresponding to a plasma frequency ℏ ω p =9.01 eV. For the hydrodynamic parameter β for Ag we employ v F =1.39 × 10 6 ms −1 . The interband permittivity ɛ inter for Ag is obtained from ref. 62 . In the SC-HDM we fix (rather than fit) the distance parameter at d =1 Å, which is of the order of the aforementioned distances between the first plane of nuclei and the edge of the jellium background [58] . By contrast, for the HW-HDM we take d to vanish, because the free electrons do not spill into the free space in this case [13] . 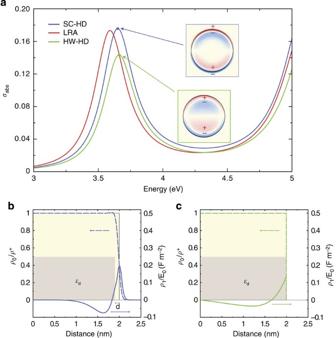Figure 3: Optical response of an Ag cylindrical nanowire of radiusR=2 nm. (a) Absorption cross-sectionσabsversus photon energy in the LRA (red line), the HW-HDM (green line) and the SC-HDM (blue line). The insets show the charge density distributionsρ1(r) at their respective dipolar SPR frequencies for the SC-HDM (blue box) and the HW-HDM (green box). (b) SC-HDM: equilibrium electron charge densityρ0normalized to the ion charge densityρ+(dashed line) and induced charge densityρ1normalized to the perturbing field amplitudeE0for the dipolar SPR, as a function of the distance from the axis of the nanowire. The light yellow shaded area indicates the jellium background profile. The grey shaded area indicates the extension of the effective polarizable medium describing the optical response of 4dcore electrons. (c) As panel (b), now for the HW-HDM. Figure 3a shows the absorption cross-sections for the Ag nanowire, computed for the same three models as for the Na nanowire in Fig. 1 . But this time for Ag both the HW- and the SC-HD models exhibit blueshifts with respect to the local-response surface-plasmon resonance at ℏ ω res =3.594 eV. In particular, in the HW-HDM the resonance occurs at ℏ ω res =3.664 eV (that is, blueshifted by 0.0697, eV), while for the SC-HDM the resonance is at ℏ ω res =3.653 eV (a blueshift of 0.0592, eV). As for Na, the difference in the peak values of the absorption cross-section can be intuitively explained as a fingerprint of the distinct geometrical cross-sections of the scatterers in the three models. Figure 3: Optical response of an Ag cylindrical nanowire of radius R =2 nm. ( a ) Absorption cross-section σ abs versus photon energy in the LRA (red line), the HW-HDM (green line) and the SC-HDM (blue line). The insets show the charge density distributions ρ 1 ( r ) at their respective dipolar SPR frequencies for the SC-HDM (blue box) and the HW-HDM (green box). ( b ) SC-HDM: equilibrium electron charge density ρ 0 normalized to the ion charge density ρ + (dashed line) and induced charge density ρ 1 normalized to the perturbing field amplitude E 0 for the dipolar SPR, as a function of the distance from the axis of the nanowire. The light yellow shaded area indicates the jellium background profile. The grey shaded area indicates the extension of the effective polarizable medium describing the optical response of 4 d core electrons. ( c ) As panel ( b ), now for the HW-HDM. Full size image While the blueshift in the HW-HDM is due to the ‘spill-in’ of the electron density inside the metal, the blueshift in the SC-HDM is a more complicated affair, related to the interplay between the 4d and 5s-band electrons at the metal–air interface: the induced charge density that contributes to the SPR oscillates at the unscreened plasma frequency in the vacuum region and it oscillates at the screened plasma frequency inside the metal. This complex mechanism leads to a net increase of the resonance frequency for Ag nanowires [58] . Our important point here is that the SC-HDM is the first semi-classical model to account for this mechanism. Figure 3b shows the equilibrium electron charge density ρ 0 for Ag nanowires, exhibiting both the charge spill-out effect and an onset of Friedel oscillations, quite analogous to the case of Na. The induced charge density ρ 1 is also shown, and although for Ag it is screened by the polarization effects of the effective medium due to interband transitions, at least up to a distance d away from the jellium interface, we again see an oscillation in the internal region, and a peak followed by decay in the free-space region. Figure 3c shows the constant equilibrium electron charge density ρ 0 and the induced charge density ρ 1 in the HW-HDM. Both are fully localized inside the nanowire, consistent with the hard-wall assumption. The charge density oscillation is due to the screening effects of the core electrons, in contrast to the monotonous spatial decay of ρ 1 for Na in Fig. 1c . Finally, a comparison of Figs 1a and 3a shows that the absorption cross-section of Ag nanowires increases for higher energies, while it drops for Na nanowires. The difference can be attributed to the interband transitions in Ag that have no counterpart in Na. The interband transitions also prevent the occurrence of a Bennett resonance in Ag nanowires. Size-dependent frequency shifts Until now we studied the SPR shifts for both Na and Ag nanowires with a fixed radius of R =2 nm, but to support our interpretations we will now present a systematic study of the dependence of the SPR shifts on the radius of the nanowire. An advantage of our semi-classical SC-HDM is that numerical calculations are feasible also for nanowires of considerably larger radii. For the HW-HDM in the quasi-static approximation, analytical espressions are known for the size-dependent resonance shift, which in that model is always a blueshift, with a leading 1/ R scaling (refs 63 , 64 ). We are now in the position to test whether this scaling behaviour is a consequence of the hard-wall approximation or also occurs in our SC-HDM that allows spill-out of the free electrons. 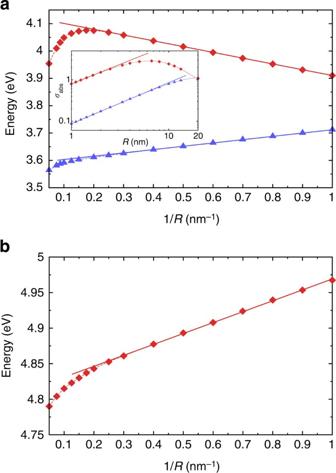Figure 4: Size-dependent SPRs shifts for Na and Ag nanowires. (a) Surface-plasmon resonance frequency versus the inverse radius 1/Rfor a Na nanowire (red squares) and an Ag nanowire (blue triangles) as calculated in the SC-HDM. The dashed lines are guides to the eye, whereas the full lines illustrate the 1/Rdependence. Inset: log–log graphs of the absorption cross-section exactly at the SPR versus radiusRfor a Na nanowire (red squares) and an Ag nanowire (blue triangles) in the LRA model. (b) ‘Bennett’ resonance frequency versus the inverse radius 1/Rfor a Na nanowire. Figure 4a shows the SPR frequency shift as a function of the inverse radius 1/ R as computed with the SC-HDM. The red line represents the data for Na. For particles of radius R <5 nm, the resonance frequency varies linearly with 1/ R , with a negative slope of −0.2 eV nm, in other words the SPR frequencies redshift when the particle size is decreased. This finding based on our SC-HDM agrees with the numerical results obtained by Li et al . [65] , who also predict the 1/ R scaling by using TD-DFT methods. Figure 4: Size-dependent SPRs shifts for Na and Ag nanowires. ( a ) Surface-plasmon resonance frequency versus the inverse radius 1/ R for a Na nanowire (red squares) and an Ag nanowire (blue triangles) as calculated in the SC-HDM. The dashed lines are guides to the eye, whereas the full lines illustrate the 1/ R dependence. Inset: log–log graphs of the absorption cross-section exactly at the SPR versus radius R for a Na nanowire (red squares) and an Ag nanowire (blue triangles) in the LRA model. ( b ) ‘Bennett’ resonance frequency versus the inverse radius 1/ R for a Na nanowire. Full size image The blue line in Fig. 4a shows the R -dependent frequency shift for Ag. This time the resonance frequency increases linearly with 1/ R for nanowire radii R <8 nm, with slope 0.12 eV nm. Thus our SC-HDM predicts that the SPR frequencies for Ag blueshift when decreasing the particle size, in agreement with the 1/ R scaling observed experimentally by Charlé et al . [66] So from Fig. 4a we can now appreciate that the 1/ R scaling is not a consequence of the hard-wall approximation, since it is now also found in the SC-HDM that includes electron spill-out. Our major result is of course our hydrodynamic (SC-HDM) prediction of the redshift for Na nanowires in Fig. 4a , where the HW-HDM incorrectly predicts a blueshift [20] , [21] (not shown here). It is important to notice that Fig. 4a shows a substantial deviation from the 1/ R dependence for Na already starting for R >5 nm, which we attribute to retardation. A similar but smaller deviation from the 1/ R scaling for Ag can also be observed in Fig. 4 , but its onset occurs for slightly larger radii, namely for R >8 nm. To substantiate our claim that the deviations from the 1/ R scaling in our SC-HDM are due to retardation, we also present LRA calculations of the dependence of the SPR peak value for σ abs on the particle radius. In the quasi-static regime this peak value follows a power-law distribution [67] , σ abs ∝ R k , which on a log–log plot as in the inset of Fig. 4 would give a straight line of slope k. The clear deviation from such power-law behaviour already for Na nanowires of radii <10 nm illustrates that the effects of the retardation become important for rather thin plasmonic nanowires also in the LRA. Nanowire radii of at least tens of nanometres are more typical in nanoplasmonic experiments. The main panel in Fig. 4 thus also nicely illustrates that the SC-HDM combines two important features: first, it describes free-electron nonlocal response and spill-out, leading to 1/ R size-dependent blueshifts for some metals and redshifts for others; second, it takes retardation fully into account, which for larger nanowires redshifts surface-plasmon resonances away from their quasi-static values. Finally, we consider the Bennett resonance frequency shift as a function of the inverse radius 1/ R as computed with the SC-HDM ( Fig. 4b ). For particles of radius R <4 nm, the resonance frequency varies linearly with 1/ R , with a positive slope of 0.14 eV nm, that is, the Bennett resonance frequencies blueshift when the particle size is decreased. Optical response of sodium and silver nanospheres Until now we have considered the optical response of cylindrical nanowires, that are translationally invariant in the axis direction, and can be treated numerically as 2D structures. In this section we will present the results obtained from the analysis of 3D structures, namely Na and Ag nanospheres both of radius R =1.5 nm. In both cases we consider the same material parameters as employed in the previous sections for Na and Ag and the same plane-wave perturbation with amplitude E 0 =1 V m −1 is assumed as well. The definition of the absorption cross-section has been adapted to the 3D case by including the sphere surface as normalization factor, that is, . The results for the Na nanosphere are shown in Fig. 5 , where the absorption cross-section of the Na nanosphere obtained with the SC-HDM is contrasted to the HW-HDM and LRA results. The dipolar SPR within the LRA occurs at ℏ ω res =3.397 eV, while it occurs at ℏ ω res =3.670 eV in the HW-HDM. This corresponds to a blueshift of 0.273 eV. For the SC-HDM the dipolar resonance appears at ℏ ω res =3.203 eV, in other words it is redshifted by 0.194 eV with respect to the LRA. So just like for the Na nanowire in Fig. 1 , we find that the HW-HDM and the SC-HDM predict opposite frequency shifts for nanospheres. And again for the SC-HDM we find a pronounced Bennett resonance, here at ℏ ω res =4.026 eV. Our neglection of Landau damping overestimates the visibility of this resonance, as our comparisons of the SC-HDM with published TD-DFT spectra for Na nanospheres in the Supplementary Fig. 3 also illustrate. 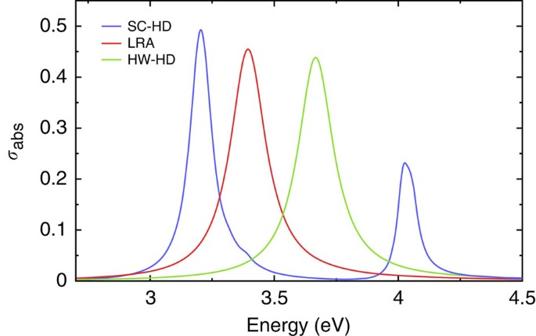Figure 5: Absorption cross-section versus photon energy for a Na nanosphere of radiusR=1.5 nm. LRA (red line), HW-HDM (green line) and SC-HDM (blue line). Figure 5: Absorption cross-section versus photon energy for a Na nanosphere of radius R =1.5 nm. LRA (red line), HW-HDM (green line) and SC-HDM (blue line). Full size image In Fig. 6 we consider the absorption cross-section of the Ag nanosphere. In particular, in the HW-HDM the resonance occurs at ℏ ω res =3.733 eV (that is, blueshifted by 0.150 eV), while for the SC-HDM the resonance is at ℏ ω res =3.721 eV (a blueshift of 0.138 eV). As for 2D calculations, the difference in the peak values of the absorption cross-section can be intuitively explained as a fingerprint of the distinct geometrical cross-sections of the scatterers in the three models. And just like for the Ag nanowires, for nanospheres the HW-HDM and the SC-HDM agree on the direction of the frequency shift as compared with the LRA, but not exactly on its magnitude. 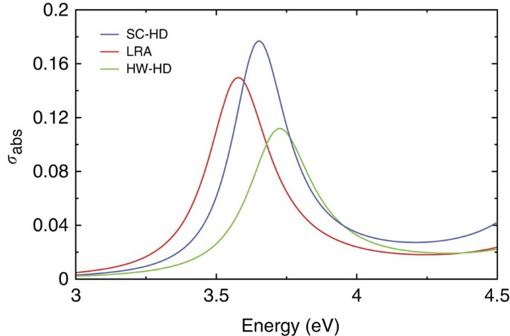Figure 6: Absorption cross-section versus photon energy for an Ag nanosphere of radiusR=1.5 nm. LRA (red line), HW-HDM (green line) and SC-HDM (blue line). Figure 6: Absorption cross-section versus photon energy for an Ag nanosphere of radius R =1.5 nm. LRA (red line), HW-HDM (green line) and SC-HDM (blue line). Full size image In conclusion, we have shown that the SC-HDM is able to describe not only nonlocal response but also electronic spill-out of both noble (Ag) and simple (Na) metals. Both the signs and the values of the resonance shifts obtained with this method agree with experimental results and predictions obtained with ab initio methods. For a decreasing particle size the SPR blueshift for Ag versus the redshift for Na are only a consequence of different well-known parameters: Drude parameters, Fermi velocities, interband permittivities ɛ ( ω ) and the spacing d between the jellium edge and the first plane of nuclei. Moreover, Bennett resonances could be identified here for the first time in a semi-classical model. We also systematically studied the size dependence of the Bennett resonance, which we believe has not been done before by other methods. We found that the Bennett resonance frequencies for Na blueshift when the particle size is decreased. The SC-HDM was obtained by extending state-of-the-art hydrodynamic models considered in nanoplasmonic research to consistently include gradients of the density into the energy functional that governs the semi-classical dynamics. Thus the inability of previous hydrodynamic models to find redshifts of SPRs for nanoparticles consisting of simple metals cannot be held against hydrodynamic models as such. Rather, it was a consequence of using too simple energy functionals that neglected the terms involving gradients of the electron density, terms which become important near metal–dielectric interfaces, being most pronounced for Na while spectrally of minor importance for Ag and Au nanowires and nanospheres. Moreover, the SC-HDM includes the effects of retardation, that are not treated in TD-DFT, unless more complicated schemes are adopted [68] . It provides a fast, flexible and reliable tool that gives the exciting possibility to treat electronic spill-out and nonlocal response in relatively large-size systems of arbitrary shapes that are of interest in nanoplasmonic applications. Think for example of large dimers with small gap sizes. For Ag nanowires and nanospheres we find quite good agreement between plasmonic resonances in the SC-HDM and in the simpler HW-HDM that neglects spill-out, justifying the use of the simpler model when not focusing on spill-out. We maintain that this good agreement for Ag (and the not so good agreement for Na) found here is not fortuitous. Rather, the agreement becomes systematically better for metals with higher work functions. Our main goal has been to develop a versatile hydrodynamic theory and numerical method that account for both retardation and electronic spill-out. Here we have shown how this can be done in a transparent and self-consistent approach, where both the static and the linear-response fields are solutions of the same energy functional. We have not tried to be as accurate as possible by fitting density-functional parameters either to experimentally measured values or to more microscopic calculations. For example, one could add fitting functions to the energy functional, fit them for a simple geometry and use them for more complex geometries. Indeed there is plenty of room to obtain even better agreement with more advanced theories. But exactly by not doing such fits, the good agreement that we already find here is exciting and promising. In the future we will employ our SC-HDM to other more complex geometries. While in the present work we have mainly focused on size-dependent frequency shifts, we envisage that in the future this model can be extended to also include size-dependent damping [69] mechanisms such as Landau damping [34] . Functional employed in the calculations The kinetic energy functional in equation (9) has already been specified in equation (10). Here we specify the XC energy functional, that we calculate by means of the LDA Gunnarson–Lundqvist functional [45] where the exchange functional is given by the Dirac term and the correlation functional is defined as The quantity is Where E h =4.35974417 10 −18 J is the Hartree energy. The dimensionless variable x is given by , where a 0 is the Bohr radius, a 0 =5.2917721092 10 −11 m. The functional derivative that appears in equation (2) is given by: where we have included the van Leeuwen and Baerends (LB94) XC-potential [48] , that provides NLDA corrections for long-range effects to the term . The functional derivative of the Thomas–Fermi functional is given by and the functional derivative of the von Weizsäcker functional is The derivative of the Dirac term is given by while the derivative is given by The van Leeuwen and Baerends (LB94) potential is where and β =0.05. Boundary conditions The HW-HDM requires an additional boundary condition at metal–dielectric interfaces, namely that the normal component of the free-electron current density should vanish. By contrast, our SC-HDM does not require additional boundary conditions at metal–dielectric interfaces. The hydrodynamic flow described by equations (2) and (3) extends over the entire 3D space. However, for a finite-size metallic object close to the origin, the confining effect of the background potential V back causes the electron fluid to extend over a finite domain surrounding the metallic structure. Thus, the density at rest n 0 ( r ) should vanish at infinity, The total density n ( r , t )= n 0 ( r )+ n 1 ( r , t ) must tend to the unperturbed density at infinity [70] , so the first-order density n 1 ( r , t ) must satisfy This condition can be rewritten for the variable ρ 1 ( r , ω ) as How to cite this article: Toscano, G. et al . Resonance shifts and spill-out effects in self-consistent hydrodynamic nanoplasmonics. Nat. Commun. 6:7132 doi: 10.1038/ncomms8132 (2015).